Unique features of the m6A methylome inArabidopsis thaliana Recent discoveries of reversible N 6 -methyladenosine (m 6 A) methylation on messenger RNA (mRNA) and mapping of m 6 A methylomes in mammals and yeast have revealed potential regulatory functions of this RNA modification. In plants, defects in m 6 A methyltransferase cause an embryo-lethal phenotype, suggesting a critical role of m 6 A in plant development. Here, we profile m 6 A transcriptome-wide in two accessions of Arabidopsis thaliana and reveal that m 6 A is a highly conserved modification of mRNA in plants. Distinct from mammals, m 6 A in A. thaliana is enriched not only around the stop codon and within 3′-untranslated regions, but also around the start codon. Gene ontology analysis indicates that the unique distribution pattern of m 6 A in A. thaliana is associated with plant-specific pathways involving the chloroplast. We also discover a positive correlation between m 6 A deposition and mRNA abundance, suggesting a regulatory role of m 6 A in plant gene expression. N 6 -methyladenosine (m 6 A) is the most prevalent internal messenger RNA (mRNA) modification [1] , [2] , [3] in eukaryotes including mammals [4] , plants [5] , [6] , Drosophila [7] and yeast [8] , as well as viruses with a nuclear phase [9] . This modification is installed by N 6 -adenosine methyltransferase. A 70 kDa SAM (S-adenosylmethionine)-binding subunit methyltransferase-like 3 (METTL3, also called MT-A70) was identified as one component of a methyltransferase complex in mammalian cells [10] . Recent studies have characterized this complex, which consists of METTL3, methyltransferase-like 14 (METTL14) and Wilms tumor 1-associated protein (WTAP) [11] , [12] , [13] . METTL14 and METTL3 are two active methyltransferases that form a heterodimer to catalyze m 6 A RNA methylation, while WTAP interacts with this complex and substantially affects the mRNA methylation inside cells but not in vitro [11] . Knockdowns of these methyltransferases affect mouse embryonic stem cell differentiation [12] . Since 2011, two m 6 A RNA demethylases of FTO and ALKBH5 have been discovered; these demethylases are involved in mammalian development, RNA metabolism and fertility [14] , [15] . These findings reveal the first examples of reversible RNA modification and indicate regulatory functions of reversible m 6 A methylation on mRNA and certain non-coding RNAs that contain m 6 A [16] . Subsequent profiling of m 6 A distributions in mammalian transcriptomes [17] , [18] and the recent mapping of the yeast m 6 A methylome in the meiotic state [19] further confirm the dynamic nature of m 6 A modification. These studies revealed that m 6 A is enriched around the stop codon and at 3′-untranslated regions (UTRs), as well as in long internal exons and at the transcription start site [17] , [18] , [19] . Cellular proteins have also been found to preferentially bind m 6 A-containing RNA [17] , [20] . The human YTH domain family 2 (YTHDF2) has recently been characterized to specifically recognize m 6 A-methylated mRNA and accelerate the decay of the bound mRNA [20] . In Arabidopsis thaliana , the m 6 A content in mRNA varies across tissues with a high ratio of m 6 A/A found in flower buds [6] . This variation correlates with the expression levels of the plant methyltransferase MTA (the plant homologue of human METTL3, encoded by At4g10760 ) [6] . Previous studies have also shown that m 6 A predominantly locates at the 3′ end of transcripts in a region 100–150 bp before the poly(A) tail in A. thaliana mRNA [21] . Inactivation of MTA prevents the progression of the developing embryo from passing the globular stage; an embryo-lethal phenotype with seed arrestment has been observed [6] . Reduced expression of MTA in A. thaliana leads to decreased m 6 A level in mRNA and abnormal growth with reduced apical dominance, abnormal organ definition and increased trichome branching [21] . These data demonstrate that m 6 A in mRNA plays a functional role in plant development. To further investigate the functions of m 6 A and to facilitate future studies of m 6 A in plants, we report here transcriptome-wide m 6 A profiling in two accessions of A. thaliana , Can-0 and Hen-16. These accessions are wild-collected natural lines from the two extremes of the natural range of photosynthetically active radiation (PAR) in the spring [22] . We show that m 6 A is a highly conserved RNA modification in mRNA across these two accessions. Intriguingly, m 6 A in A. thaliana is enriched not only around the stop codon and within 3′ UTRs, as in yeast and mammalian systems, but also around the start codon, a property distinct from other known m 6 A methylomes [17] , [18] . A positive correlation between m 6 A deposition and mRNA levels indicates a regulatory role of m 6 A in plant gene expression. m 6 A is abundant and conserved in A. thaliana mRNA m 6 A is known to be a relatively abundant internal modification in A. thaliana mRNA [6] . 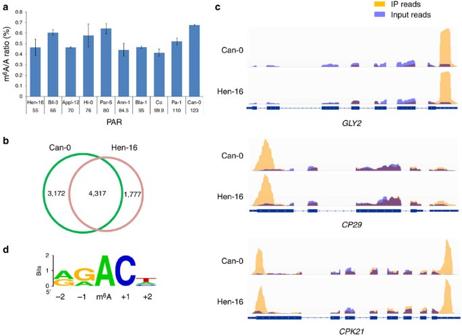Figure 1: Overview of m6A methylome inA. thaliana. (a) The m6A/A ratio of mRNA isolated from eachA.thalianastrain. Error bars are calculated as the s.d. from three replicates. PAR values are displayed below the strain names. (b) Numbers of strain-specific and common m6A peaks. (c) Examples of m6A peaks conserved between Can-0 and Hen-16. Orange colour represents IP reads, while blue colour represents input reads. The purple colour comes from mixing orange with blue. (d) The RRACH conserved sequence motif for m6A-containing peak regions. We selected ten geographically diverse accessions of A. thaliana to grow in a common laboratory environment to measure the m 6 A/A ratio of purified mRNA ( Supplementary Table 1 ). These wild-collected natural lines were collected from sites that vary widely in PAR values [22] . We observed that the ratio of m 6 A/A in total mRNA from these ten accessions varied within the range of 0.45–0.65% ( Fig. 1a ), although not in direct relation to PAR, suggesting that the m 6 A methylation level in mRNA is relatively stable but potentially affected by complex environmental factors. Figure 1: Overview of m 6 A methylome in A. thaliana . ( a ) The m 6 A/A ratio of mRNA isolated from each A . thaliana strain. Error bars are calculated as the s.d. from three replicates. PAR values are displayed below the strain names. ( b ) Numbers of strain-specific and common m 6 A peaks. ( c ) Examples of m 6 A peaks conserved between Can-0 and Hen-16. Orange colour represents IP reads, while blue colour represents input reads. The purple colour comes from mixing orange with blue. ( d ) The RRACH conserved sequence motif for m 6 A-containing peak regions. Full size image To obtain the transcriptome-wide m 6 A map of whole A. thaliana plants, we interrogated two accessions (Can-0 and Hen-16) using the m 6 A-targeted antibody coupled with high-throughput sequencing [17] , [18] . Can-0 was originally collected from the Canary Islands where PAR in spring is 123.74, the highest seen for 1,191 accessions of A. thaliana [22] . Hen-16 was obtained from northern Sweden where spring PAR is 55.29 (ref. 22 ), the lowest end of the range. The m 6 A level in mRNA isolated from Can-0 is higher than that from Hen-16 as measured by LC-MS/MS ( Fig. 1a ). More than 70% of the m 6 A peaks of Can-0 and Hen-16 were consistently detected in two biological replicates for each accession. We used these recurrent peaks as high-confidence m 6 A sites for further analysis. In total, we identified 7,489 m 6 A peaks representing the transcripts of 6,289 genes in Can-0, and 6,094 m 6 A peaks representing transcripts of 5,416 genes in Hen-16 ( Supplementary Data 1 ). Among them, 4,317 m 6 A peaks were detected within both Can-0 and Hen-16 ( P <1e−5, Chi-squared test), indicating that m 6 A is highly conserved across A. thaliana accessions ( Fig. 1b,c , Supplementary Data 1 ). We validated 11 m 6 A peak-containing genes by PCR with quantitative reverse transcription (RT–qPCR) and all of them showed significant enrichment in immunoprecipitation (IP)-pull-down samples ( Supplementary Fig. 1 ). 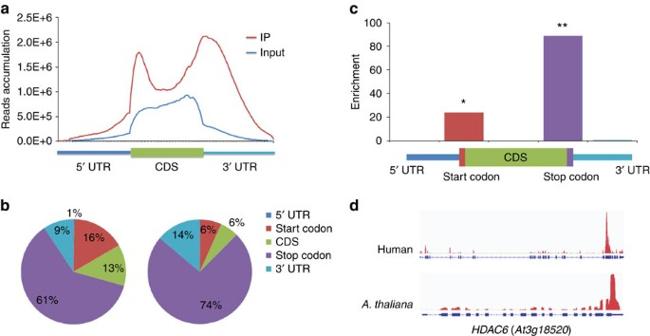Figure 2: Distribution pattern of m6A peaks along transcripts. (a) Accumulation of m6A-IP reads along transcripts. Each transcript is divided into three parts: 5′ UTRs, CDs and 3′ UTRs. (b) The m6A peak distribution within different gene contexts. Left panel: total genes with m6A peaks; right panel: genes conserved in human andArabidopsis. (c) The m6A peak distribution along a metagene. Enrichment scores are calculated as;n, number of peaks belonging to each category;N, number of total peaks;p, proportion of each category within the genome by length. *P<2.2e−16, **P<1e−30.Pvalues are determined by Chi-squared test. (d) An example of homologous genes with m6A peaks conserved in human andA. thaliana. CDs, coding regions. On the basis of these results, we estimated that the A. thaliana transcriptome contains 0.5–0.7 m 6 A peaks per 1,000 nucleotides or 0.7–1.0 m 6 A peaks per actively expressed transcript ( Supplementary Table 2 , Supplementary Fig. 2 ). These levels are comparable with those obtained in mammals [17] . The relative abundance of m 6 A peaks in mRNAs from Can-0 and Hen-16 is consistent with total m 6 A levels measured in mRNAs isolated from these two accessions ( Fig. 1a,b ). To determine if the m 6 A peaks that we identified contained the m 6 A consensus sequence of RRACH (where R represents purine, A is m 6 A and H is a non-guanine base) [23] , [24] , we analyzed the top 1,000 most significant peaks ( Supplementary Fig. 3 ). We found at least one such motif in 934 peaks ( Fig. 1d ). The same sequence motif appears to be necessary for m 6 A methylation in plant mRNA as it has been observed in mammals and yeast mRNA ( Supplementary Fig. 4 ) [17] , [18] , [19] . m 6 A distribution exhibits a distinct topology in A. thaliana We next analyzed the distribution of m 6 A in the whole transcriptome for both strains of A. thaliana . We determined the distribution of m 6 A reads along transcripts in the m 6 A-IP and non-IP (input) samples, respectively. Intriguingly, we found that the reads from m 6 A-IP are highly enriched around the start codon, stop codon and within 3′ UTRs in both strains ( Fig. 2a and Supplementary Fig. 5 ). The prevalence of m 6 A-IP reads around the start codon has not been observed in mammals or yeast. Figure 2: Distribution pattern of m 6 A peaks along transcripts. ( a ) Accumulation of m 6 A-IP reads along transcripts. Each transcript is divided into three parts: 5′ UTRs, CDs and 3′ UTRs. ( b ) The m 6 A peak distribution within different gene contexts. Left panel: total genes with m 6 A peaks; right panel: genes conserved in human and Arabidopsis . ( c ) The m 6 A peak distribution along a metagene. Enrichment scores are calculated as ; n , number of peaks belonging to each category; N , number of total peaks; p , proportion of each category within the genome by length. * P <2.2e−16, ** P <1e−30. P values are determined by Chi-squared test. ( d ) An example of homologous genes with m 6 A peaks conserved in human and A. thaliana . CDs, coding regions. Full size image To further confirm the preferential locations of m 6 A on transcripts, we investigated the metagene profiles of m 6 A peaks. Consistent with the distribution of reads, m 6 A peaks are abundant near the stop codon (61%) and start codon (16%), followed by the coding regions (13%) and then 3′ UTRs (9%) ( Fig. 2b ). After segment normalization by the total length of each gene portion, we observed that m 6 A is exclusively enriched around the start codon and stop codon ( Fig. 2c ). We mapped the number of m 6 A peaks around the start codon, the stop codon and upstream of transcription termination site ( Supplementary Fig. 6a–c ). The m 6 A peaks are enriched at three locations: the region 60 bp downstream and 50 bp upstream of the start codon, the region 80 bp downstream and 100 bp upstream of the stop codon and the region 80–220 bp before the poly(A) tail; the last location of enrichment is consistent with the previous finding that m 6 A preferentially locates at the 3′ end of transcripts in a region 100–150 bp before the poly(A) tail in Arabidopsis [21] . We focused on the m 6 A peaks near the start codon and identified several new sequence motifs by comparing peak regions with scrambled background sequences, suggesting the possibility that distinct sequence motifs may exist for m 6 A methylation in plant mRNA ( Supplementary Fig. 7 ). Using strict criteria of peptide similarity, we identified 1,684 m 6 A-containing transcripts/genes in A. thaliana that are conserved in humans. Through comparison with the published data [17] , we found that 813 of these transcripts (48%) are also methylated in humans ( Supplementary Data 2 ). Interestingly, almost all of the conserved methylated sites are located at the stop codon (74%) and 3′ UTRs (14%) of transcripts ( Fig. 2b,d ), thus highlighting that m 6 A peaks around the start codon are specific to A. thaliana . We depicted the m 6 A peak distribution along transcripts in available data sets of human and mouse, confirming the observation that m 6 A is exclusively enriched at the stop codon and 3′ UTRs in these systems ( Supplementary Fig. 8 ). Clearly, the enrichment of m 6 A near the start codon in A. thaliana is distinct. This feature of the m 6 A distribution may play a unique role in plant-specific pathways. m 6 A-containing mRNAs in important biological pathways The presence of m 6 A is critical for normal plant development [6] , [21] . To uncover further functional insights about m 6 A in A. thaliana , we selected genes containing m 6 A in both Can-0 and Hen-16 and identified the enriched gene ontology (GO) terms using the DAVID tool. We found that these genes are highly enriched in chloroplast/plastid and protein transport/localization categories ( Fig. 3a ). 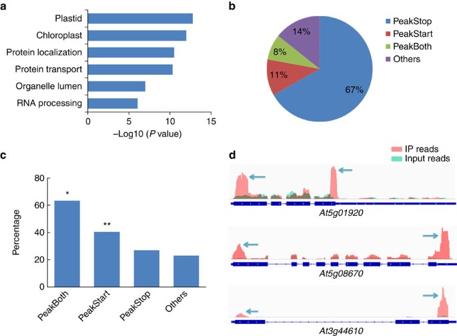Figure 3: Functional annotation of genes with m6A. (a) GO-enrichment analysis of all the genes with m6A peaks. GO categories are maintained by Gene Ontology Consortium.Pvalues are calculated using the DAVID tool. (b) Percentages of subgroups of genes divided by the position pattern of m6A peaks. (c) Percentages of genes characterized as chloroplast related for each subgroup. *P<6.0e−25 (PeakBoth), **P<5.2e−18 (PeakStart).Pvalues are calculated using the DAVID tool. (d) Examples of chloroplast genes with m6A peaks at both the start and stop codon. The m6A-IP peaks are indicated by arrows. Figure 3: Functional annotation of genes with m 6 A. ( a ) GO-enrichment analysis of all the genes with m 6 A peaks. GO categories are maintained by Gene Ontology Consortium. P values are calculated using the DAVID tool. ( b ) Percentages of subgroups of genes divided by the position pattern of m 6 A peaks. ( c ) Percentages of genes characterized as chloroplast related for each subgroup. * P <6.0e−25 (PeakBoth), ** P <5.2e−18 (PeakStart). P values are calculated using the DAVID tool. ( d ) Examples of chloroplast genes with m 6 A peaks at both the start and stop codon. The m 6 A-IP peaks are indicated by arrows. Full size image We next sought to determine if the unique m 6 A position patterns are related to plant-specific GO categories. We classified genes into four subgroups according to the distribution of m 6 A peaks: PeakStart (m 6 A peaks around start codon), PeakStop (m 6 A peaks around stop codon), PeakBoth (m 6 A peaks around both start and stop codons) and others ( Fig. 3b and Supplementary Data 1 ). Then we performed GO-enrichment analysis for each subgroup. All subgroups of m 6 A-containing genes exhibit high enrichment of chloroplast-related cellular components, indicating that a large proportion of these genes produce proteins localized in chloroplast though encoded by nuclear genome ( Supplementary Fig. 9 ). Strikingly, >60% of genes belonging to the PeakBoth subgroup could be attributed to chloroplast components ( Fig. 3c ). Similarly, about 40% of the genes belonging to the PeakStart subgroup are associated with chloroplast. Photosynthesis is one of the most important functions in plants; 10–20% of nuclear genes encode proteins that are imported to chloroplast [25] . Apparently, genes with m 6 A enrichment around the start codon are highly enriched in chloroplast components. The significant enrichment of chloroplast-related GO categories among transcripts with m 6 A peaks around the start codon prompted us to examine photosynthesis-related genes in PeakStart and PeakBoth subgroups. Indeed, we identified dozens of well-studied photosynthesis-related genes that carry m 6 A peaks ( Supplementary Data 3 ). For instance, At5g01920 (or STN8) is an important chloroplast thylakoid protein kinase that is specific to the phosphorylation of N-terminal threonine residues in D1, D2 and CP43 proteins and Thr-4 in PsbH of the photosystem II [26] . In our m 6 A-IP data, the transcript of STN8 contains two clear m 6 A peaks around the start and stop codons ( Fig. 3d ). The large fraction of m 6 A-containing genes associated with chloroplast suggests a relationship between m 6 A mRNA methylation and photosynthesis, one of the defining processes of plants. Strain-specific m 6 A marking of mRNAs Although most m 6 A peaks are shared between the two A. thaliana strains, we could detect a proportion of strain-specific peaks, even using strict criteria (Methods). In total, we identified 1,319 Can-0-specific peaks and 546 Hen-16-specific peaks ( Supplementary Data 4 ). Furthermore, some of the common m 6 A peaks in these two strains showed altered intensity ( Fig. 4 ). GO analysis indicated that the genes with dynamic m 6 A peaks are enriched in several categories of fundamental biological functions including mRNA metabolic process, response to stimulus and regulation of translational elongation ( Supplementary Data 5 ). For instance, At5g06290 (or 2-Cys Prx B ) has been shown to be sensitive to light intensities and oxidative stress [27] . In our m 6 A-IP data, we observed significant m 6 A peaks around the start codon of At5g06290 in Can-0 but not in Hen-16 ( Fig. 4 ). 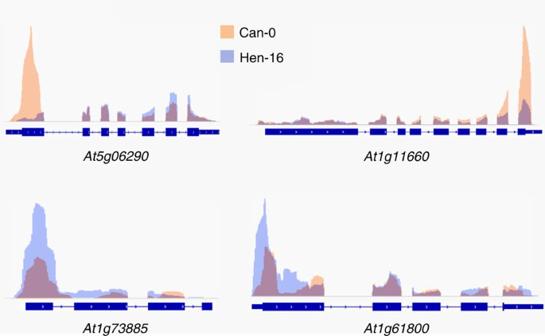Figure 4: Dynamic m6A peaks in twoArabidopsisstrains. Different colours illustrate the accumulation of m6A-IP reads from two accessions. Figure 4: Dynamic m 6 A peaks in two Arabidopsis strains. Different colours illustrate the accumulation of m 6 A-IP reads from two accessions. Full size image As an initial exploration into the functional implications of m 6 A methylation differences across genomes, we asked whether m 6 A methylation could underlie expression differences. Using the RNA-Seq data, we calculated gene expression to assign differentially expressed genes (DE genes) of the two strains. Indeed, we found 801 more highly expressed genes in Can-0 (Can-high) and 1,011 more highly expressed genes in Hen-16 (Hen-high) ( Fig. 5a and Supplementary Data 6 ), perhaps reflecting, at least in part, the substantial differences in PAR in the native habitat of these accessions. Within the Can-high list, we detected many more genes that contained m 6 A peaks in Can-0 than in Hen-16 (195/81, P <0.01, Fisher’s exact test). Correspondingly, in the list of Hen-high genes, we detected more genes containing m 6 A peaks in Hen-16 than in Can-0 (221/140, P <0.01, Fisher’s exact test) ( Fig. 5a ). This observation suggests that each strain possesses its own characteristic m 6 A methylation sites that appear to be associated with gene activation. This hypothesis seems to contradict the recent discovery that a main function of m 6 A is to mediate mRNA degradation in mammalian cells [11] , [12] , [13] , [20] . However, when we checked positions of the m 6 A peaks involved in upregulated genes, we found that a large portion of these peaks are located at the 5′ end of the corresponding DE genes ( Supplementary Data 6 ). To confirm this observation, we divided strain-specific m 6 A-containing genes into two groups and examined how their expression levels correlate with the locations of m 6 A peaks. Our analysis showed that m 6 A peaks at the 5′ end of transcripts correlate with higher expression levels of each strain. Genes in the PeakStart category possesses higher overall expression levels and correlate well with strain-specific m 6 A peaks ( Fig. 5b , note that the gene expression ratios of Can-0/Hen-16 are shown). We further examined the fraction of each subgroup of genes based on their expression levels. Genes with both 5′- and 3′-m 6 A peaks (PeakBoth) are enriched in the high-expression fraction, while genes with m 6 A peaks at other locations (PeakOther) tend to be lower expressed ( Fig. 5c ). Thus, m 6 A enrichment at the 5′ end of the plant transcripts correlates with higher expression level in A. thaliana in general, perhaps by stabilizing the transcripts via reader proteins or interaction with translation machineries. 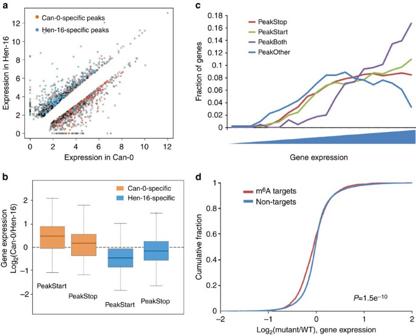Figure 5: Relationship between m6A peaks and mRNA level. (a) Differentially expressed mRNAs in Can-0 and Hen-16. Genes with Can-0-specific m6A peaks are highlighted in orange and genes with Hen-0-specific m6A peaks are highlighted in blue. (b) The ratio of mRNA expression levels in two samples containing strain-specific m6A peaks. Genes are divided into two categories (PeakStart and PeakStop) according to the peak positions. (c) Fraction of genes belonging to each subgroup defined by the m6A distribution pattern. Genes are sorted by expression levels. (d) Cumulative distribution of mRNA expression changes between themtamutant and WT for m6A-modified genes (red) and non-target genes (blue).Pvalues are calculated by two-sided Mann–Whitney test. WT, wild type. Figure 5: Relationship between m 6 A peaks and mRNA level. ( a ) Differentially expressed mRNAs in Can-0 and Hen-16. Genes with Can-0-specific m 6 A peaks are highlighted in orange and genes with Hen-0-specific m 6 A peaks are highlighted in blue. ( b ) The ratio of mRNA expression levels in two samples containing strain-specific m 6 A peaks. Genes are divided into two categories (PeakStart and PeakStop) according to the peak positions. ( c ) Fraction of genes belonging to each subgroup defined by the m 6 A distribution pattern. Genes are sorted by expression levels. ( d ) Cumulative distribution of mRNA expression changes between the mta mutant and WT for m 6 A-modified genes (red) and non-target genes (blue). P values are calculated by two-sided Mann–Whitney test. WT, wild type. Full size image In a recent study, Bodi et al . [21] generated an m 6 A reduction mutant of A. thaliana and profiled gene expression. They identified 883 upregulated and 654 downregulated genes in the mutant plant [21] . By comparing the DE genes with our list of m 6 A peaks, we found that 116 among 883 upregulated transcripts are modified by m 6 A, whereas 142 among 654 downregulated transcripts contain m 6 A ( Supplementary Data 7 ). These data suggest that transcripts carrying m 6 A tend to be downregulated in the m 6 A reduction mutant ( P <0.01, Chi-squared test). We extended this analysis to the whole transcriptome. Indeed, among genes with m 6 A modification, more are downregulated than upregulated in the m 6 A reduction mutant plant. This trend did not exist for genes without m 6 A modification ( Fig. 5d ). Together, their data supported our hypothesis that m 6 A tends to positively correlate with gene expression in a large fraction of transcripts in A. thaliana . Mammalian microRNA (miRNA)-binding sites are mostly found within 3′ UTRs [28] ; however, in plants they occur typically in the coding regions of target transcripts [29] . Unlike mammals, miRNAs in plants recognize the target sites by near-perfect sequence complementarity. By comparing the transcripts containing m 6 A with the public miRNA targets database (TAIR) [30] , we found that only 5% of known miRNA-targeted transcripts contain m 6 A. Furthermore, we employed a de novo miRNA target prediction method [31] to inspect m 6 A peak regions. Among the top 1,000 most significant m 6 A peak regions, only 11 regions could be potentially targeted by miRNA ( Supplementary Data 8 ). Taken together, our results indicate that m 6 A is unlikely to directly impact miRNA binding sites in A. thaliana , although such an association has been proposed in animals [18] . However, we could not exclude the possibilities that m 6 A may affect miRNA maturation, or impact miRNA targeting sites through reader proteins of m 6 A or structural changes induced by methylation. The discovery of m 6 A demethylases and the mapping of the m 6 A methylomes in mammalian systems indicate that m 6 A methylation of mRNA is a reversible and dynamic process with regulatory functions [14] , [15] , [16] , [17] , [18] , [32] , [33] . The importance of m 6 A in post-transcriptional regulation of gene expression is further reinforced by the discovery and characterization of mammalian reader proteins that recognize m 6 A modifications of mRNA and subsequently affect the stability of the target transcripts [20] . Previous studies have shown that m 6 A plays a critical role in plant development [6] , [21] . Here, we report the transcriptome-wide m 6 A distributions in two accessions of A. thaliana , Can-0 and Hen-16. We found that m 6 A is highly conserved across A. thaliana accessions. The methylation sites in a portion of transcripts are also conserved in corresponding transcripts of humans, indicating a fundamental functional role of m 6 A in eukaryotes. Nevertheless, there are differences between the two A. thaliana accessions with a higher total m 6 A level in Can-0 than Hen-16, and with ~1,400 more m 6 A peaks identified in Can-0. The m 6 A distribution could be influenced by differences in the accession’s climates of origin and genetic backgrounds. The modification sites could be conserved but the modification fraction at each site could vary depending on environmental factors. Importantly, we discovered features of the m 6 A distribution in A. thaliana mRNA that are distinct from those of mammals: (i) m 6 A in both accessions is enriched around the stop codon and at 3′ UTRs, as it has been found in mammals, but also around the start codon; (ii) the m 6 A methylation around the start codon is heavily associated with the chloroplast, a photosynthesis organelle in plants. In addition, m 6 A is less likely to be directly associated with miRNA recognition sites in A. thaliana . These distinct differences, namely the start codon enrichment of m 6 A and its association with chloroplast, strongly suggest additional, plant-specific functions of this mRNA methylation. Previous studies indicated that the currently available m 6 A antibody could also recognize N 6 ,2′-O-dimethyladenosine (m 6 Am) [17] , [19] , which might lead to enrichment peaks at transcription start site. However, in our results, the start codon enrichment is clearly distinct from the m 6 Am peak observed previously [17] ( Fig. 1 ). More accurate, base-resolution methods are highly desirable to determine the exact sites and modification fractions in the future. Noticeably, the distinct enrichment of m 6 A around the start codon correlates with the overall upregulation of mRNA expression level. This relationship contradicts observations in mammalian systems, in which m 6 A methylation around the stop codon and at 3′ UTRs is negatively correlated with gene expression [11] , [12] , [20] . Published microarray data using a different accession of Arabidopsis (Col-0) also supports our findings with high correlations with our RNA-seq data ( Supplementary Fig. 10 ) [21] . Although our analysis demonstrates significant overlap of m 6 A sites between the two ecotypes (Can-0 and Hen-16), more precise analysis would benefit from future studies on coincident accessions. Our results suggest that m 6 A reader proteins may exist in A. thaliana to recognize m 6 A at the 5′ end and subsequently affect the stability of the target mRNA. This function could directly impact translation through the methylation itself or through the reader protein(s). It should be noted that several RNA-binding proteins have been pulled down as potential ‘m 6 A readers’ with a few biochemically confirmed to specifically recognize methylated mRNAs [17] , [20] . In particular, YTHDF2 has been shown to bind and accelerate the decay of m 6 A-modified mRNA [20] . However, the functions of other m 6 A readers are still unknown; some of them could promote translation of a specific set of transcripts. Our discovery suggests the versatile roles of m 6 A in plants beyond mediating mRNA decay. It has been demonstrated that m 6 A methyltransferase in A. thaliana is critical for normal plant development [6] , [21] . We found that the transcripts with m 6 A are highly enriched in chloroplast/plastid and protein transport/localization categories, indicating a mechanism by which m 6 A affects plant-specific metabolism. Past studies have demonstrated that light and circadian cycles impact the stability and translation of specific plant transcripts [34] , [35] , [36] , [37] . However, the mechanisms of post-transcriptional gene regulation in response to light availability have not been clearly understood. The stability and translation of chloroplast mRNAs are known to be regulated by RNA-binding proteins that reside at 5′ and 3′ UTRs [38] . Intriguingly, our data show that >60% of mRNAs containing m 6 A at both the start and stop codons encode proteins that could be components of the chloroplast ( Fig. 3c ). Given that 10–20% of nuclear-encoded genes are associated with the chloroplast and photosynthesis in plant [25] , this percentage represents a significant enrichment. It is possible that the dynamic m 6 A methylation at 5′ and 3′ ends modulate the RNA affinities of RNA-binding proteins, thereby controlling mRNA transport and localized expression. Though technologies that can provide more accurate measurements of the m 6 A sites are required in the future to gain deeper insights (for example, splicing), the first m 6 A transcriptome-wide map of a plant species A. thaliana presented here provides a starting roadmap for uncovering m 6 A functions that may affect/control plant metabolism in the future. Plant material Seeds from the Can-0 and Hen-16 accessions of A. thaliana were sown in 50:50 Metromix 200:Farfad C2 soil in 48-cell flats and stratified for 5 days at 4 °C to synchronize germination. Seedlings were germinated in controlled-environment growth chambers at the University of Chicago greenhouses on a 16-hour light and 8-hour dark cycle. Plants were thinned between days 5 and 7 of growth. Above-ground tissue was harvested between the fifth and seventh hour of the light cycle on day 21. The tissue was flash frozen in liquid nitrogen, ground using a mortar and pestle and stored at −80 °C. High-throughput m 6 A sequencing To obtain sufficient (10 mg) total RNA for IP of m 6 A-containing mRNA, ~200 plants from each accession were harvested and pooled in 0.6 and 2.1 g quantities. RNA was extracted using a protocol modified from a published procedure [39] ; reactions took place in 15 or 50 ml conicals, and reagents were scaled up linearly with respect to the increased tissue mass, with 20 or 70 times the amount of each reagent, respectively. RNA was tested for quality via Nanodrop and gel electrophoresis. Polyadenylated RNA was extracted using FastTrack MAG Maxi mRNA isolation kit (Invitrogen). RNA was randomly fragmented to ~200 nt by RNA Fragmentation Reagents (Ambion). Fragmented RNA was incubated for 2 h at 4 °C with m 6 A antibody (Synaptic Systems Cat. No. 202003, diluted to 0.5 μg μl −1 ) in IP buffer (50 mM Tris-HCl, 750 mM NaCl and 0.5% Igepal CA-630) supplemented with BSA (0.5 μg μl −1 ). The mixture was then incubated with protein-A beads and eluted with elution buffer (1 × IP buffer and 6.7 mM m 6 A). Eluted RNA was precipitated by 75% ethanol. The eluted RNA was treated with RNasin (Ambion Cat No. AM2694) according to the manufacturer’s instructions. TruSeq Stranded mRNA Sample Prep Kit (Illumina) was used to construct the library from immunoprecipitated RNA and input RNA according to a published protocol [40] . Sequencing was done on an Illumina HiSeq machine with 2 × 100 cycles Solexa paired-end sequencing. RT–qPCR validation for m 6 A-enriched genes Eleven genes enriched in the m 6 A-IP and six genes not differentially expressed between the IP and non-IP samples were tested by RT–qPCR. Data cleanup and analysis proceeded as described by previous protocol [41] . The dissociation curves for each reaction were plotted and those with irregular features were removed. RNA passed through a beads only column, which should not bind any RNA, was treated as the input control for the IP step. Ct values from qPCR on the flow-through from the m 6 A-IP and the m 6 A-IP were expressed as the percent input of the beads only sample. Primer sequences are listed in Supplementary Data 9 . Detailed information for plotting the qPCR figure can be found in an online manual at: http://www.lifetechnologies.com/us/en/home/life-science/epigenetics-noncoding-rna-research/chromatin-remodeling/chromatin-immunoprecipitation-chip/chip-analysis.html. Data analysis Sequence data were analyzed according to the procedure described by Meyer et al . [18] Briefly, Tophat [42] with Bowtie [43] was run to align the input and IP-sequenced samples to the Columbia reference genome and annotation file (Tair10) [30] . The BEDTools tool [44] was used to divide the aligned accepted hits into 1 bp intervals. The read depth was then averaged for each 25 nt discrete, non-overlapping genomic window using an ad hoc R program ( Supplementary Data 10 ). To identify 25 nt windows enriched for m 6 A, the number of reads that mapped to each window for the IP and input sample, and the total reads for each, were compared using Fisher’s exact tests and corrected for multiple testing using Benjamini–Hochberg to reduce false discovery rate to 0.05. To determine which of these windows cluster to form distinct peaks, we concatenated adjacent significant windows together and filtered out peaks <100 nt in length. Significant peaks with false discovery rate <0.05 in Can-0, Hen-16 or both were annotated using an ad hoc R script ( Supplementary Data 10 ). IntersectBED with the Columbia reference genome and annotation file was used to further annotate this set of significant peaks [44] . Peaks that shared >50% overlapping length were defined as recurrent peaks. For a peak to be classified as strain specific, it should not overlap (one nucleotide) any peak in any two replicates of the other strain. Sequence motifs were identified by using Homer [45] . Gene expression was calculated by Cufflinks [42] using the input-sequencing reads. Cuffdiff [42] was used to find the DE genes between Can-0 and Hen-16. Gene function analysis (GO enrichment) was performed with the DAVID tool [46] . Plant miRNA targets were predicted by psRobot [31] . Microarray data were downloaded from GEO (accession ID: GSE349243) and RMA method [47] was introduced to calculate gene expression and DE genes between mta mutant and wide type. How to cite this article: Luo, G.-Z. et al . Unique features of the m 6 A methylome in Arabidopsis thaliana . Nat. Commun. 5:5630 doi: 10.1038/ncomms6630 (2014). Accession codes: The high-throughput data used in this study are deposited in the NCBI GEO database with accession number GSE59154 .